Control superstructure of rigid polyelectrolytes in oppositely charged hydrogels via programmed internal stress Biomacromolecules usually form complex superstructures in natural biotissues, such as different alignments of collagen fibres in articular cartilages, for multifunctionalities. Inspired by nature, there are efforts towards developing multiscale ordered structures in hydrogels (recognized as one of the best candidates of soft biotissues). However, creating complex superstructures in gels are hardly realized because of the absence of effective approaches to control the localized molecular orientation. Here we introduce a method to create various superstructures of rigid polyanions in polycationic hydrogels. The control of localized orientation of rigid molecules, which are sensitive to the internal stress field of the gel, is achieved by tuning the swelling mismatch between masked and unmasked regions of the photolithographic patterned gel. Furthermore, we develop a double network structure to toughen the hydrogels with programmed superstructures, which deform reversibly under large strain. This work presents a promising pathway to develop superstructures in hydrogels and should shed light on designing biomimetic materials with intricate molecular alignments. Hydrogels are a class of soft and water-containing material. Recent developments of tough hydrogels [1] , [2] , [3] have greatly expanded the applications of this material in various fields, including soft actuators, artificial organs, regenerative medicine, and so on [4] , [5] , [6] , [7] , [8] , [9] . Beyond the toughness, one of the next challenges is how to introduce macroscale superstructures into isotropic and amorphous hydrogels. Many specific functions of biological tissues are strongly related to the superstructures of rigid, fibre-forming molecules. For example, collagen fibres in the articular cartilage align parallel to the sliding surface but perpendicular to the interface with bone [10] , [11] , [12] . These superstructures of collagen fibres are considered important for the functions of cartilages, including low sliding friction and strong bonding to the bone [13] , [14] , [15] . These natural systems with spatially intricate superstructures provide us elegant paradigms in designing new biomimetic materials with specific functions and promising applications. However, developing programmable macroscale superstructure in hydrogels is a non-trivial aim because the bottom-up approach of self-assembly no longer works. Many efforts have been made to induce uniaxial polymer orientation in hydrogels, for example, by shear, electric or magnetic fields [16] , [17] , [18] , [19] , [20] , [21] . These methods are not straightforwardly applicable to develop complicated macroscale superstructure in the hydrogels, and alternative strategies are definitely required. Herein, we report a novel strategy to develop hydrogels with macroscale superstructures from rigid fibre-forming molecules by playing with programmed internal stress. When a soft hydrogel has a swelling mismatching in different regions, an internal stress develops. The internal stress can direct orientation of rigid fibre-forming molecules. In this work, we applied photolithographic technology to induce programmed swelling mismatching in the positively charged hydrogel ( Fig. 1a ) [22] , [23] . Considering a slab of hydrogel with alternative stripes of different swellings, the large swelling region experiences a compression from the less swelling region. Oppositely, the less swelling region experiences an extension from the large swelling region. If rigid rod-like molecules are embedded in the hydrogel matrix, they intend to orient along the tensile direction while they orient perpendicular to the compressive direction ( Fig. 1b ). This internal-stress-directed orientation of rigid molecules inside the hydrogels has recently been demonstrated [24] , [25] , [26] . When both of the embedded rigid macromolecules and the hydrogels are polyelectrolytes but carry opposite charges, the orientation can be ‘memorized’ by polyion complex formation by the dialysis of their counterions [25] , [26] . Therefore, various superstructures of rigid polyelectrolytes could be developed in oppositely charged polymeric hydrogels by harnessing internal-stress-directed orientation of rigid macromolecules. By using double network concept [1] , we further developed tough double network hydrogels with programmed superstructures. This work gives a pathway to synthesize tough hydrogels with complex superstructure and should merit designing other biomimetic materials towards specific functions. 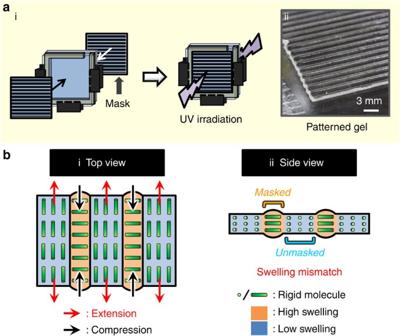Figure 1: Photolithographic patterned hydrogels with controllable swelling mismatch and resulting internal-stress-directed orientation of rigid macromolecules. (a) Experimental set-up for synthesis of programmed superstructure in the hydrogels using photolithographic method. As an example, two identical photo masks of stripe pattern are placed in phase on two surfaces of the reaction cell containing precursor solution of gel (i). The width of masked regions (black) and unmasked regions (white) is 2 and 0.6 mm, respectively. UV was irradiated from both sides of the cell to initiate polymerization. After gelation, the as-prepared gel shows morphology characteristic to the mask pattern (ii). (b) Schematic to show the built-up of internal stress because of the swelling mismatch, and the resultant superstructure of rigid molecules in the photolithographic patterned gels. In the gel, composition gradient between the masked and unmasked regions leads to swelling mismatch. For stripe-patterned hydrogel, as shown ina, the large swelling region experiences a compression from the less swelling region. Rigid molecules embedded in the gel intend to orient along the tensile direction while they orient perpendicularly to the compressive direction. Thus, the patterned swelling mismatch induces programmed internal stress, which directs the orientation of the rigid macromolecules. Using oppositely charged rigid molecules and polymer network, the structure is memorized by polyion complex formation after dialysis of their counterions. Figure 1: Photolithographic patterned hydrogels with controllable swelling mismatch and resulting internal-stress-directed orientation of rigid macromolecules. ( a ) Experimental set-up for synthesis of programmed superstructure in the hydrogels using photolithographic method. As an example, two identical photo masks of stripe pattern are placed in phase on two surfaces of the reaction cell containing precursor solution of gel (i). The width of masked regions (black) and unmasked regions (white) is 2 and 0.6 mm, respectively. UV was irradiated from both sides of the cell to initiate polymerization. After gelation, the as-prepared gel shows morphology characteristic to the mask pattern (ii). ( b ) Schematic to show the built-up of internal stress because of the swelling mismatch, and the resultant superstructure of rigid molecules in the photolithographic patterned gels. In the gel, composition gradient between the masked and unmasked regions leads to swelling mismatch. For stripe-patterned hydrogel, as shown in a , the large swelling region experiences a compression from the less swelling region. Rigid molecules embedded in the gel intend to orient along the tensile direction while they orient perpendicularly to the compressive direction. Thus, the patterned swelling mismatch induces programmed internal stress, which directs the orientation of the rigid macromolecules. Using oppositely charged rigid molecules and polymer network, the structure is memorized by polyion complex formation after dialysis of their counterions. Full size image Superstructure formation in hydrogel We use poly(2,2′-disulfonyl-4,4′-benzidine terephthalamide) (PBDT), a polyanion, as the rigid macromolecule, and chemically crosslinked poly( N -[3-( N,N -dimethylamino)propyl] acrylamide methyl chloride quaternary) (PDMAPAA-Q), a polycation network, as the hydrogel. The chemical structures of these two polymers are shown in Fig. 2 . 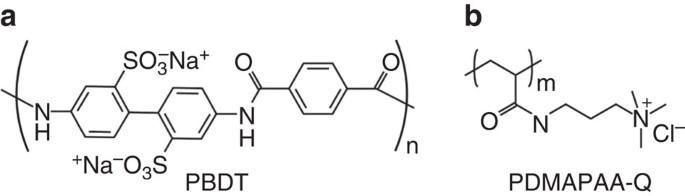Figure 2: Chemical structure of components. (a) The rigid anionic polyelectrolyte, PBDT, which is embedded in hydrogel matrix. (b) The flexible cationic polyelectrolyte, PDMAPAA-Q, which forms a hydrogel network by chemically crosslinking. Figure 2: Chemical structure of components. ( a ) The rigid anionic polyelectrolyte, PBDT, which is embedded in hydrogel matrix. ( b ) The flexible cationic polyelectrolyte, PDMAPAA-Q, which forms a hydrogel network by chemically crosslinking. Full size image The gel with superstructure was synthesized by polymerizing the precursor aqueous solution containing prescribed amount of the rigid polyanion PBDT, cationic monomer DMAPAA-Q, chemical cross-linker and photo initiator (see Methods). Two identical photo masks of stripe pattern were placed in phase on the surfaces of the reaction cell, composed of two pieces of glass plates separated by a silicone spacer of 1 mm in thickness, to guide the photo-initiated polymerization and gelation process, which built a composition gradient in the gel ( Fig. 1a ). It took 7.5 h to finish the gelation in both the masked and unmasked regions and to obtain an integrated piece of gel strong enough for handling. The as-prepared gel was transparent with a periodical groove pattern of thickness undulation, where thin parts were located in the middle of masked regions, as shown in Fig. 3a (top view) and Fig. 3b (side view). The boundary of the thin parts and thick parts did not coincide with that of the mask, but inside the masked region, 0.7 mm from the masking boundary, because of the non-parallel irradiation of the UV light and the diffusion of reactive species during the reaction (see Supplementary Fig. 1 and Supplementary Table 1 ). For simplicity, however, we called the thin part as the masked region and the thick part as the unmasked region in the later text. Under polarizing optical microscope (POM), the sample showed strong birefringence in masked regions, as observed from top of the sample ( Fig. 3aii ). However, when observed from cross-section of the sample, the central layer of unmasked regions showed birefringence ( Fig. 3bii ). The birefringence of the gel comes from both PBDT that has a positive birefringence and PDMAPAA-Q that has a negative birefringence. Previous study has shown that PBDT has a much stronger birefringence than PDMAPAA-Q, and the net birefringence observed here is related to the orientation of the rigid PBDT molecules [25] , [26] , [27] . From the birefringence colour observed with 530-nm-sensitive tint plate ( Fig. 3aiii, biii , ), we identified that PBDT aligns parallel to the stripes in the masked regions ( Fig. 3aiv ) and aligns parallel to the gel surface, yet without in-plane directional preference in the central layer of unmasked regions ( Fig. 3biv ). As the gel was synthesized at a PBDT concentration (1 wt%) lower than its critical liquid crystalline concentration ( C LC *=2.8 wt%), this result indicates that internal stress built during the gelation directs the orientation of PBDT. During the synthesis of sheet-shape gel by photopolymerization, both surface layers of the sample have a faster reaction speed, resulting in composition gradient in the gel thickness direction. The gelation at the central layer is relatively slow to freeze the complexation process, which leads to localized volume contraction to some extent. As a result, the central layer of the gel is stretched by the surface layers, and PBDTs align along with the stretching stress, that is, parallel to the gel surface. 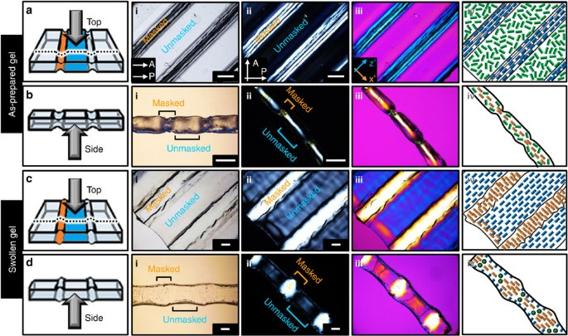Figure 3: Characterization of superstructure formed in patterned hydrogels. Observation of superstructure of PBDT in patterned PDMAPAA-Q hydrogels at as-prepared (a,b) and swollen (c,d) states. The gels were observed under POM from top (a,c) and side (b,d) directions. The thickness of the observation direction from side was unified into ~2 mm. The images in column (i) were observed under the parallel polarizers, columns (ii) and (iii) were observed under the crossed polarizers without and with 530-nm tint plate, respectively. The column (iv) is a schematic illustration of the orientation of PBDT molecules within the gel, where the green bars represent PBDTs with weak orientation, the green circles represent PBDTs orientation of vertical direction to the sheet, the orange and blue bars represent highly ordered PBDTs. A: Analyzer; P: Polarizer; X′: fast axis of the tint plate; Z′: slow axis of the tint plate. Scale bar, 1 mm. Figure 3: Characterization of superstructure formed in patterned hydrogels. Observation of superstructure of PBDT in patterned PDMAPAA-Q hydrogels at as-prepared ( a , b ) and swollen ( c , d ) states. The gels were observed under POM from top ( a , c ) and side ( b , d ) directions. The thickness of the observation direction from side was unified into ~2 mm. The images in column (i) were observed under the parallel polarizers, columns (ii) and (iii) were observed under the crossed polarizers without and with 530-nm tint plate, respectively. The column (iv) is a schematic illustration of the orientation of PBDT molecules within the gel, where the green bars represent PBDTs with weak orientation, the green circles represent PBDTs orientation of vertical direction to the sheet, the orange and blue bars represent highly ordered PBDTs. A: Analyzer; P: Polarizer; X′: fast axis of the tint plate; Z′: slow axis of the tint plate. Scale bar, 1 mm. Full size image After swelling, the masked regions had a higher swelling ability than the unmasked region. Both the regions showed strong birefringence, yet with different colours, indicating the different orientations of PBDT, as illustrated in Fig. 3c . The PBDT in the masked regions oriented vertical to the stripes’ direction while it oriented parallel to the stripes’ direction in the unmasked regions. The alignment of PBDT was also confirmed by side view of the samples ( Fig. 3d and Supplementary Fig. 2 ). We should notice that the birefringence of masked regions changed from blue of as-prepared gel to orange of the swollen gel ( Fig. 3a,c ), indicating a reversion of PBDT alignments. This reversion of PBDT orientation is related to the change of the internal stress field by the swelling. Before swelling, the thicknesses of the masked and unmasked regions of the as-prepared gels were 0.7 and 0.9 mm, respectively. Thus, the masked regions, having a low swelling ability, experience a tension from the unmasked regions ( Fig. 3b ). As a result, the PBDT molecules in the masked regions aligned parallel to the boundary. However, after swelling, the masked regions have a higher swelling ability than the unmasked region ( Fig. 3d ). Therefore, this region receives a compression along the boundary and PBDT molecules convert the orientation to the direction perpendicular to the boundary. On the other hand, the unmasked region, which has less swelling ability, receives a tension along the boundary that directs the PBDT molecules to align with this tensile direction. The gel shows a global anisotropic swelling, with slightly large swelling in the direction vertical to the stripes. The swelling of the hydrogel in pure water removes the paired small counterions of the oppositely charged polyelectrolytes from the gel matrix (dialysis effect), and, therefore, the orientation of PBDT directed by internal stress in the hydrogel was ‘memorized’ by polyion complex formation. As the polymer matrix is in excess of its mass than that of the PBDT, a large ionic osmotic pressure still exists to swell the gel substantially. We confirmed that the superstructure was maintained even after releasing of the internal stress by slicing the masked and unmasked regions into separate stripes ( Supplementary Fig. 3 ). In addition to the POM observation, we also characterized the localized molecular alignments in the gels using linear dichroism measurements; PBDT alignments extracted from the LD results matched well with those from POM ( Supplementary Fig. 4 ). We should note that, although the patterned gels showed strong birefringence, PBDT only possesses weak orientation, as revealed by the small linear dichroic ratio ( Supplementary Fig. 4 ). For simplicity and better understanding the proposed mechanism, however, we drawn the PBDT in perfect alignments in the schematic figures. The swelling mismatching depends on many factors, such as the dimension of mask, the polymerization kinetics, the formulation of the precursor solution of gel, and so on. In the present system, the swelling mismatching boundary was not sharply coincident with the mask boundary but located inside the mask region, 0.7 mm from the boundary. Therefore, when the width of the masked region was decreased below a value of 1.5 mm, strong swelling mismatching could not be formed, and we observed a decrease in the birefringence of unmasked regions. The detailed relationship between the swelling mismatching and experimental conditions should be reported in a forthcoming paper. Universality for creating complex superstructures Following the above concept, hydrogels with more complex superstructures could be developed by designing different masks to control the swelling mismatching ( Fig. 4 ). We used three basic shapes, stripe, dot and branch as masked regions (black) to build five mask patterns with different features. Besides the periodical straight stripes (mask I) as already shown in Fig. 1 , concentric circle stripes (mask II), periodical cubic dots (mask III), hexagonal dots (mask IV) and periodical honey-comb networks (mask V) were designed ( Fig. 4 , top). These mask patterns can be classified into three types: (A) line symmetric (I), (B) circular symmetric (II) and (C) periodical (III, IV, V). 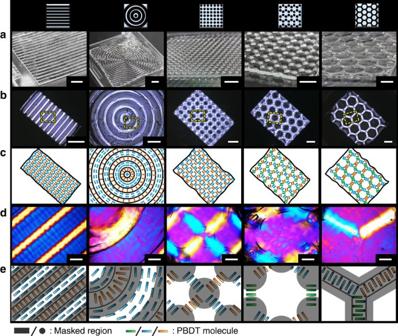Figure 4: Controlling of superstructure in hydrogels by using different masks. (a) Images of the as-prepared gels taken by digital camera to show the gel appearances and patterns. The masks used for photolithography are shown in the top of each column, where the masked regions are black and unmasked regions are white. Scale bar, 5 mm. (b) Images of swollen gels observed under circular polarized light. The oriented domains show strong birefringence. Scale bar, 1 cm. (d) The yellow rectangle regions shown in row (b) were observed by crossed polarizers with 530-nm tint plate to determine the molecular orientation. Scale bar, 1 mm.c,eSchematic illustrations of the orientation of PBDT molecules within the swollen gel, where the orange, blue and green bars represent highly ordered orientation. The grey regions inecorrespond to the regions of masks, where the central parts of gels have high swelling. Size of mask patterns: (I) width of masked stripes and distance between stripes are 1.5 and 0.5 mm, respectively. (II) Width of masked stripes and distance between stripes are 2.0 and 0.6 mm, respectively. (III,IV) Diameter of dots and distance between dots are 2.0 and 0.6 mm, respectively. (V) Width and length of branch line are 1.5 and 4.0 mm, respectively. Figure 4: Controlling of superstructure in hydrogels by using different masks. ( a ) Images of the as-prepared gels taken by digital camera to show the gel appearances and patterns. The masks used for photolithography are shown in the top of each column, where the masked regions are black and unmasked regions are white. Scale bar, 5 mm. ( b ) Images of swollen gels observed under circular polarized light. The oriented domains show strong birefringence. Scale bar, 1 cm. ( d ) The yellow rectangle regions shown in row ( b ) were observed by crossed polarizers with 530-nm tint plate to determine the molecular orientation. Scale bar, 1 mm. c , e Schematic illustrations of the orientation of PBDT molecules within the swollen gel, where the orange, blue and green bars represent highly ordered orientation. The grey regions in e correspond to the regions of masks, where the central parts of gels have high swelling. Size of mask patterns: (I) width of masked stripes and distance between stripes are 1.5 and 0.5 mm, respectively. (II) Width of masked stripes and distance between stripes are 2.0 and 0.6 mm, respectively. (III,IV) Diameter of dots and distance between dots are 2.0 and 0.6 mm, respectively. (V) Width and length of branch line are 1.5 and 4.0 mm, respectively. Full size image The as-prepared gels with these masks also showed grooves or wells in the masked regions ( Fig. 4a ). After the gels were swelled in water, the masked regions showed higher swelling ratio than the unmasked regions. The swelling mismatch led to programmed strong internal stress and PBDT alignments, which were confirmed by observation under circular polarizing light ( Fig. 4b ). The alignments of PBDTs identified by POM images with tint plate ( Fig. 4d ) for swollen gels are illustrated in Fig. 4c,e . Type (A) has been discussed in the previous text; here we consider type (B). The mask of circular stripes produces circular orientation of PBDT in the unmasked region that experiences a tension because of less swelling, and radial orientation in the masked region that experiences a compression due to more swelling ( Fig. 4 , Column II), similar to the effect of the straight stripe mask ( Fig. 4 , Column I). The gel also showed a global saddle-like deformation, indicating that the outer region of the gel swells more than that of the inner region, and a net internal stress leads to the deformation of the gel [28] . Then, we consider type (C). The dot mask (cubic dots and hexagonal dots) produces dot-like high swelling regions ( Fig. 4 , Columns III, IV). In these cases, the unmasked regions between two nearest dots experience compression in the direction of line that connects the two dots. As a result, the PBDT molecules in this region oriented perpendicular to the line that connects the two dots. Since the stress in the centre of the cubic or hexagonal patterns is cancelled, PBDT has no preferential orientation in the central region. The honey-comb mask produces network-like high swelling regions ( Fig. 4 , Column V). Since these network arms are under compression, PBDT molecules oriented perpendicular to the network arms. PBDT has no preferential orientation in the central region of the network, indicating that there is no net stress in this region. Thus, all the gels of type (C) share the common feature that the internal stress is cancelled in the centre of unmasked region to give amorphous structure in this region. These gels, having no net stress globally, were flat after swelling. These results demonstrate that by designing proper masks, very complicated liquid crystal domains are possible to be obtained. Toughening the superstructure hydrogels As common polyelectrolyte hydrogels, these superstructure hydrogels were mechanically weak. Taking advantage of their polyelectrolyte nature, we further toughen these gels by introducing a second neutral network, based on the double network concept [1] , [29] ( Supplementary Fig. 5 ). The superstructures were preserved even after inducing the second network of polyacrylamide ( Fig. 5a,b ). The obtained double network gel was much tougher than its single network, sustaining large tensile deformation. Accompanying with the deformation, the superstructure deformed reversibly without rupture ( Fig. 5a,b ). The tensile stress–strain curves are anisotropic, showing higher fracture stress and strain along the strip direction than those of the vertical direction ( Fig. 5c ). These anisotropic mechanical properties should be attributed to the patterned gel structure itself, not to the PBDT superstructure. The movie and detailed structure change during the deformation are shown in the Supplementary Information ( Supplementary Movies 1 and 2 ). 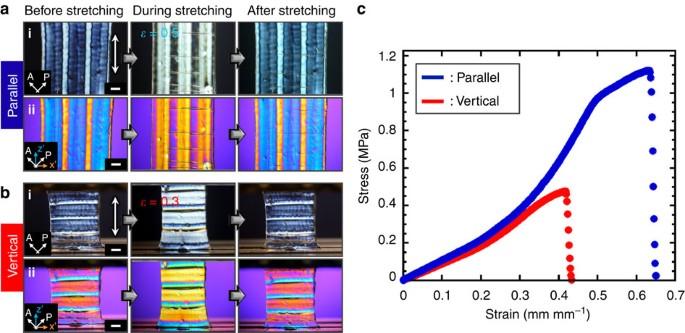Figure 5: Toughening double network hydrogels with superstructures. (a,b) Birefringence patterns showing the reversible change in the stripe superstructures of double network (DN) gel during stretching in the direction parallel (a) and vertical (b) to the strip direction. Images in rows (ai) and (bi) were observed under the crossed polarizers. Images in rows (aii) and (bii) were observed under the crossed polarizers with 530-nm tint plate. Double-headed arrow shows the tensile direction. Tensile strain,ε, is defined as (L−L0)/L0, in whichL0andLare the lengths of the gel before and during elongation, respectively. Scale bar, 2 mm. (c) Stress–strain curves of DN gels stretched in the directions parallel (blue) and vertical (red) to the stripe direction. Figure 5: Toughening double network hydrogels with superstructures. ( a , b ) Birefringence patterns showing the reversible change in the stripe superstructures of double network (DN) gel during stretching in the direction parallel ( a ) and vertical ( b ) to the strip direction. Images in rows (ai) and (bi) were observed under the crossed polarizers. Images in rows (aii) and (bii) were observed under the crossed polarizers with 530-nm tint plate. Double-headed arrow shows the tensile direction. Tensile strain, ε , is defined as ( L − L 0 )/ L 0 , in which L 0 and L are the lengths of the gel before and during elongation, respectively. Scale bar, 2 mm. ( c ) Stress–strain curves of DN gels stretched in the directions parallel (blue) and vertical (red) to the stripe direction. Full size image In conclusion, we have developed macroscale superstructure hydrogels with alignments of rigid polyelectrolyte molecules by tuning the internal stress field. By photolithographic patterning, we can programme the swelling mismatch of the gels, which induces large internal stress. This internal stress directs orientation of rigid macromolecules, which are frozen by the strong polyion complexation between the two oppositely charged polyelectrolytes. By using the double network concept, these superstructure gels can be developed into tough double network gels. At the moment, we could only prepare the superstructure gels containing low concentration of PBDT (several wt%) because of its high-viscosity limitation. Accordingly, we did not observe distinct mechanical property or swelling property originated from this superstructure. In future, we will apply this idea to rigid biomolecules with relatively low molecular weight at high concentration for creation of specific functions. For example, by controlling the orientation of rigid collagen molecules in tough double network hydrogels, we are able to develop hydrogels with anisotropic mechanical properties similar to cartilages. Structural biomacromolecules, such as F-actin, microtubule and collagen, are all negatively charged rigid molecules. During tissue growth, different growth rates will build internal stress that may also play a role in directing the orientation of these structural biomacromolecules. This work should give insight in understanding the structure formations of these biomacromolecules in living cells and soft tissues. Synthesis of hydrogels with programmed swelling mismatching To synthesize hydrogel film with programmed swelling mismatching, photolithographic technique was adopted. The reaction cells were prepared by sandwiching the square frame of a silicone spacer (thickness: 1 mm) between two parallel glass plates. Then, two photo masks with the same pattern prepared by colour-laser printing on Overhead projector films (OHP films;KOKUYO Co., Ltd., Japan) were gripped on two sides of the reaction cell in phase, to guide the progress of photo polymerization at specific regions ( Fig. 1c ). The aqueous precursor solutions contained 1.0 wt% of the rigid anionic polymer, PBDT (average molecular weight, M w ,=200,000 g mol −1 , see Supplementary Fig. 6 ), 2.0 M of the cationic monomer, DMAPAA-Q, 2.0 mol% of the chemical cross-linker, N,N′ -methylenebis(acrylamide) (MBAA) and 0.15 mol% of the photoinitiator, 2-oxoglutaric acid (OA). The amount in mol% was relative to the cationic monomer concentration. After proper mixing, the precursor solution was injected into the reaction cells. As-prepared gels were obtained after UV irradiation from the both sides of the reaction cell (UV light intensity was 3.9 mW cm −2 ) for 7.5 h under an argon atmosphere at room temperature. By using masks with different patterns described in Fig. 4 , gels with different programmed swelling mismatching were obtained. The as-prepared gels were swelled in a large amount of water for several days to achieve the equilibrium state. Synthesis of tough double network gels with superstructures The PBDT-containing PDMAPAA-Q gel was used as the first network, and polyacrylamide was used as the second network. The as-prepared PBDT-containing PDMAPAA-Q gel was immersed in precursor solution of the second network (4 M acrylamide monomer, 0.01mol% MBAA and 0.01mol% OA) for 2 days until reaching equilibrium. Then the second network was formed using UV irradiation for 10 h (ref. 29 ). The as-prepared double network gels were swelled in water for several days to achieve the equilibrium state. Optical observation of superstructure The surface morphology and the birefringence of the gels in the as-prepared state and the equilibrium swelling state were observed under a POM (Nikon, Eclipse, LV100POL) in the parallel and crossed polarization modes, respectively, at room temperature. Sample gels were placed on glass slides and observed from the top ( Fig. 3a,c ) or side ( Fig. 3b,d ). All the samples of PBDT-containing PDMAPAA-Q gel exhibited a first-order white-grey birefringence colour. To identify the molecular orientation direction, a 530-nm-sensitive tint plate was inserted [25] , [26] , [27] . PBDT has a positive birefringence and PDMAPAA-Q has a negative birefringence. At the prescribed condition in this study, the birefringence intensity of PBDT surpasses that of PDMAPAA-Q [24] , [25] . Therefore, the birefringence colour observed is governed by the PBDT orientation. The birefringence patterns of gels in the equilibrium swelling state were also observed under optical microscope (OLYMPUS, SZX12) with circular polarizer plate (MeCan Imageing Inc., Saitama, Japan) at room temperature. Sample gels were sandwiched between clockwise and counterclockwise circularly polarizing plates and observed from the top ( Fig. 4b ). The highly oriented parts in the patterned gel exhibited a white-grey birefringence colour regardless of the orientation direction [30] , [31] . Other experimental details are described in Supplementary Methods . How to cite this article: Takahashi, R. et al. Control superstructure of rigid polyelectrolytes in oppositely charged hydrogels via programmed internal stress. Nat. Commun. 5:4490 doi: 10.1038/ncomms5490 (2014).